Plasmon resonance enhanced multicolour photodetection by graphene Graphene has the potential for high-speed, wide-band photodetection, but only with very low external quantum efficiency and no spectral selectivity. Here we report a dramatic enhancement of the overall quantum efficiency and spectral selectivity that enables multicolour photodetection, by coupling graphene with plasmonic nanostructures. We show that metallic plasmonic nanostructures can be integrated with graphene photodetectors to greatly enhance the photocurrent and external quantum efficiency by up to 1,500%. Plasmonic nanostructures of variable resonance frequencies selectively amplify the photoresponse of graphene to light of different wavelengths, enabling highly specific detection of multicolours. Being atomically thin, graphene photodetectors effectively exploit the local plasmonic enhancement effect to achieve a significant enhancement factor not normally possible with traditional planar semiconductor materials. Graphene is emerging as an attractive material candidate for future electronics [1] , [2] , [3] and optoelectronics [4] , [5] due to its unique combination of several important characteristics, including high carrier mobility [6] , high optical transparency [7] , exceptional mechanical flexibility and strength [8] . Ultra-high speed electronic and photonic devices with the operation frequency up to terahertz regime have been demonstrated or suggested [9] , [10] , [11] , [12] , [13] , [14] . Recent studies have demonstrated the exciting potential of exploiting graphene for diverse optoelectronic devices including solar cells, touch panels, photodetectors, ultra-fast lasers, polarizer and optical modulators [15] , [16] , [17] , [18] , [19] , [20] , [21] . The wideband absorption [7] , high carrier mobility [6] and short carrier lifetime make graphene an ideal material for wideband, high-speed photodetectors. Ultra-fast metal-graphene-metal photodetectors have been demonstrated, with operation frequency (40 GHz achieved and 500 GHz suggested) comparable to or exceeding traditional group III–V materials-based photodetector [9] , [22] . Importantly, with a zero band gap, graphene photodetectors can be used for ultra-wide band (300 nm–6 μm) operation, far exceeding the capability of the current photodetectors [23] , [24] . Additionally, with the fast development in chemical vapour deposition (CVD) growth of large area graphene [25] , [26] , [27] and its exceptional mechanical flexibility [8] , graphene-based photodetectors may be implemented over large area and in a flexible form at a low cost that is not possible with traditional group III–V semiconductor-based technologies. However, the performance of graphene-based photodetectors reported to date is limited at least by two factors arising from its intrinsic characteristics. The first limitation is associated with the low photoresponsivity and very low external quantum efficiency (QE) (0.1–0.2%) [16] , [22] largely due to its intrinsically poor light absorption properties ( ∼ 2.3% for single layer graphene). Another limitation is the lack of spectral selectivity in intrinsic graphene, which is originated from the wavelength-independent absorption characteristics of graphene due to the constant universal conductivity G for Dirac fermions [7] . Although the graphene absorption characteristics can be modified in the infrared regime by tuning the Fermi level away from Dirac point [28] , [29] , the spectral selectivity achieved with this approach is, however, relatively weak with a shallow cutoff edge. To overcome these limitations and achieve overall practical advantages in graphene-based photodetectors, here we report a new strategy to fabricate highly sensitive multi-color photodetectors by integrating graphene with a thin layer of plasmonic nanostructures. Plasmonic nanostructures have been explored for surface-enhanced Raman spectroscopy of graphene [30] . We show that the plasmonic nanostructures can be prepared on a first substrate and transferred onto CVD-grown graphene without degrading its electronic performance. Here the plasmonic nanostructures can act as subwavelength scattering source and nano-antennas to enhance the optical detection and photoresponse at selected plasmon resonance frequency, and therefore enabling graphene photodetectors that respond sensitively to selected colours. Photoresponse studies show that the integration with plasmonic nanostructures can greatly enhance the photocurrent by up to 1,500%, with the external QE reaching up to ∼ 1.5% at zero source drain bias and zero gate voltage, about one order of magnitude better than previously reported graphene devices ( ∼ 0.1–0.2% at zero bias) [16] , [22] . 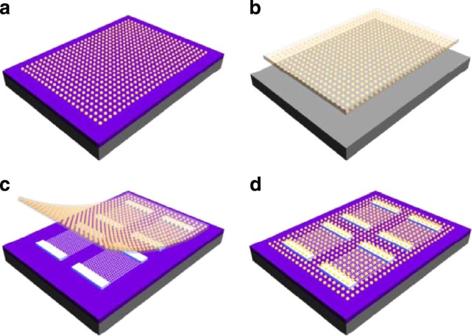Figure 1: Schematic illustration of the fabrication process to integrate plasmonic nanoparticles with graphene. (a) Gold nanoparticles are obtained by thermally annealing 4 nm thick gold film on the SiO2substrate. (b) PMMA is spin coated on the substrate, followed by a lifting-off process using buffered oxide etch to obtain free-standing PMMA/Au-nanoparticle thin film. (c) PMMA/Au-nanoparticle thin film is fished by pre-made back-gate CVD graphene transistors. (d) PMMA is dissolved away to leave gold nanoparticles on the surface of the graphene devices. Grey, blue, yellow and white represent silicon, silicon dioxide, gold nanoparticles and gold electrode, respectively. Device fabrication and characterization Figure 1 shows the schematic illustration of the process flow to couple plasmonic nanostructures with graphene devices. In general, back-gated graphene transistors are first fabricated on silicon/silicon oxide substrate using CVD-grown graphene. The coupling between the plasmonic nanostructures with graphene is accomplished through a transfer process. Specifically, a 4 nm thick gold thin film is first sputtered on a Si/SiO 2 substrate, followed by a thermal annealing process at 350 °C for 15 min under forming gas atmosphere, to result in a high density monolayer of gold nanoparticles ( Fig. 1a ). A poly(methyl methacrylate) (PMMA) layer is then spin coated onto the gold nanoparticle array to fully wrap the nanoparticles inside, followed by a lifting-off process using buffered oxide etch to obtain a free-standing PMMA/nanoparticle thin film ( Fig. 1b ). After repeated rinsing with de-ionized water to remove the buffered oxide etch residues, the PMMA/nanoparticle thin film is fished by pre-fabricated back-gate graphene transistors ( Fig. 1c ). Finally, PMMA is dissolved away to leave gold nanoparticles on the surface of the graphene devices ( Fig. 1d ). Figure 1: Schematic illustration of the fabrication process to integrate plasmonic nanoparticles with graphene. ( a ) Gold nanoparticles are obtained by thermally annealing 4 nm thick gold film on the SiO 2 substrate. ( b ) PMMA is spin coated on the substrate, followed by a lifting-off process using buffered oxide etch to obtain free-standing PMMA/Au-nanoparticle thin film. ( c ) PMMA/Au-nanoparticle thin film is fished by pre-made back-gate CVD graphene transistors. ( d ) PMMA is dissolved away to leave gold nanoparticles on the surface of the graphene devices. Grey, blue, yellow and white represent silicon, silicon dioxide, gold nanoparticles and gold electrode, respectively. Full size image Scanning electron microscopy was used to characterize the gold nanoparticle array before and after the transferring process on Si/SiO 2 surface and graphene surface, respectively ( Fig. 2a,b ). The scanning electron microscopy image of the thermally annealed gold nanoparticles on Si/SiO 2 surface ( Fig. 2a ) shows a high-density array of Au nanoparticles with an average diameter ∼ 18 nm and density of 1,320 particle per μm 2 ( Supplementary Fig. S1 ). After transferring onto the graphene devices, the gold nanoparticle array structure is well kept with nearly the same morphology ( Fig. 2b ). To investigate the plasmon resonance characteristics of these Au nanoparticle array on graphene, we transferred Au nanopartilces onto a continuous CVD graphene layer on glass substrate using the same process, with which ultraviolet-visible spectral analysis is used to study the absorption/scattering characteristics in the gold-plasmonic-nanostructure—graphene heterostructures. The extinction spectrum of the CVD graphene layer shows a nearly flat absorption of ∼ 2.3% (black line in Fig. 2c ), consistent with the expected absorption by a single layer graphene. Importantly, the nanoparticle-graphene conjugate exhibits a strong plasmon resonance enhanced absorption/extinction of nearly 21% with a pronounced resonance peak around 515 nm (red line in Fig. 2c ). 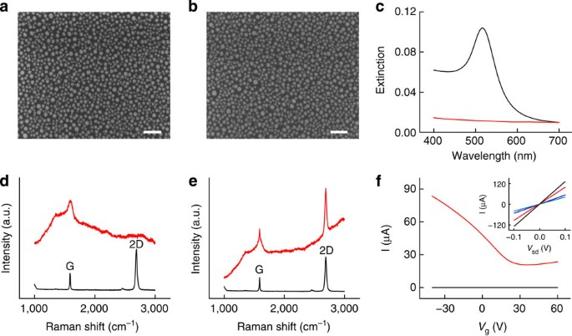Figure 2: Characterization of the graphene and graphene transistors with transferred gold nanoparticles. (a) Scanning electron microscopy (SEM) image of the gold nanoparticles obtained by annealing a Au thin film on SiO2surface at 350 °C before the transferring process. Scale bar 100 nm. (b) SEM image of gold nanoparticles transferred onto graphene surface. Scale bar 100 nm. (c) Ultraviolet-visible spectrum of graphene on glass (black line) shows a nearly flat spectrum with an absorption of∼2.3%, and that of nanoparticle/graphene (red line) on glass shows a plasmonic resonance peak around 515 nm with a peak absorption of∼21%. (d) Raman spectroscopy of the graphene (black line), and graphene with Au nanoparticles obtained by directly annealing 4 nm gold thin film on graphene (red line). The diminishing 2D peak (2,690 nm) indicates the nearly complete destruction of graphene structure by the Au deposition and annealing processes. (e) Raman spectroscopy of graphene (black line), and graphene with transferred Au nanoparticles (red line). The G peak (1,590 nm) and 2D peak (2,690 nm) is well kept in this case, demonstrating that the integrity of the graphene is preserved. (f)Transfer characteristics (I-Vg) atVd=50 mV for a back-gated graphene transistor with transferred Au nanoparticles (red line), and a graphene transistor with directly annealed Au nanoparticles (black line). The inset shows the source drain currentIversus source-drain voltageVsdof the graphene transistor with transferred Au nanoparticles at gate −20, 0, 20 and 40 V (black, red, blue and green lines), respectively. The device has a length of 8 μm and width of 8 μm. These studies demonstrate that the electrical performance of the graphene transistors is retained in the device with transferred Au nanoparticles, but not in the device with directly annealed Au nanoparticles, consistent with Raman studies. Figure 2: Characterization of the graphene and graphene transistors with transferred gold nanoparticles. ( a ) Scanning electron microscopy (SEM) image of the gold nanoparticles obtained by annealing a Au thin film on SiO 2 surface at 350 °C before the transferring process. Scale bar 100 nm. ( b ) SEM image of gold nanoparticles transferred onto graphene surface. Scale bar 100 nm. ( c ) Ultraviolet-visible spectrum of graphene on glass (black line) shows a nearly flat spectrum with an absorption of ∼ 2.3%, and that of nanoparticle/graphene (red line) on glass shows a plasmonic resonance peak around 515 nm with a peak absorption of ∼ 21%. ( d ) Raman spectroscopy of the graphene (black line), and graphene with Au nanoparticles obtained by directly annealing 4 nm gold thin film on graphene (red line). The diminishing 2D peak (2,690 nm) indicates the nearly complete destruction of graphene structure by the Au deposition and annealing processes. ( e ) Raman spectroscopy of graphene (black line), and graphene with transferred Au nanoparticles (red line). The G peak (1,590 nm) and 2D peak (2,690 nm) is well kept in this case, demonstrating that the integrity of the graphene is preserved. ( f) Transfer characteristics ( I - V g ) at V d =50 mV for a back-gated graphene transistor with transferred Au nanoparticles (red line), and a graphene transistor with directly annealed Au nanoparticles (black line). The inset shows the source drain current I versus source-drain voltage V sd of the graphene transistor with transferred Au nanoparticles at gate −20, 0, 20 and 40 V (black, red, blue and green lines), respectively. The device has a length of 8 μm and width of 8 μm. These studies demonstrate that the electrical performance of the graphene transistors is retained in the device with transferred Au nanoparticles, but not in the device with directly annealed Au nanoparticles, consistent with Raman studies. Full size image Before we developed the transfer process to couple Au nanoparticles with graphene, we have attempted to obtain Au nanoparticle array on graphene by directly evaporating an Au thin film on graphene followed by thermal annealing, which can result in similar nanoparticles. However, Raman spectrum of the graphene after this process indicates that the graphene lattice structure is severely degraded as evidenced by the diminishing 2D peak at 2,690 nm (red line in Fig. 2d ). Further electrical measurement confirms that the device is completely damaged with an open circuit (black line in Fig. 2f ). In contrast, the coupling of Au nanoparcticles with graphene through the transfer process described above retains the structure integrity of the graphene as shown by the well-kept G peak (1,590 nm) and 2D peak (2,690 nm) in Raman spectrum (red line in Fig. 2e ). Electrical measurements show that the graphene device with transferred Au nanoparticles exhibit typical gate transfer and source-drain output performance of a graphene transistors ( Fig. 2f red line and inset). The carrier mobility of the graphene devices with transferred Au nanoparticles is typically in the range of 1,000–2,000 cm 2 V −1 s −1 , comparable to those without Au nanoparticles ( Supplementary Fig. S2 ). Plasmon resonance enhanced photodetection To characterize the photoresponse characteristics of these devices, scanning photocurrent measurement was performed at zero source-drain bias and zero gate voltage, with a well-focused laser beam scanned from source to drain. The short circuit photocurrent is measured as a function of the laser position, with a resolution of ∼ 1 μm ( Fig. 3a ). The location-dependent photocurrent measurements of the graphene devices with (red line, Fig. 3b ) and without (black line, Fig. 3b ) Au nanoparticles show several important features. First, the maximal photocurrent response is observed when light is focused in the graphene channel near the graphene–metal junction. Second, the position-dependent photocurrent plot shows an anti-symmetric characteristic, in which the photocurrent generated at each electrode is opposite and the photocurrent is nearly zero at the centre of the channel. These observations suggest that the photocurrent generation is originated from the band offset near the metal-graphene contact. The antisymmetrical photocurrent in metal-graphene-metal device was also observed in previous reports [16] , [31] , and can be attributed to the nearly symmetric band structure at both contact electrodes along the device. 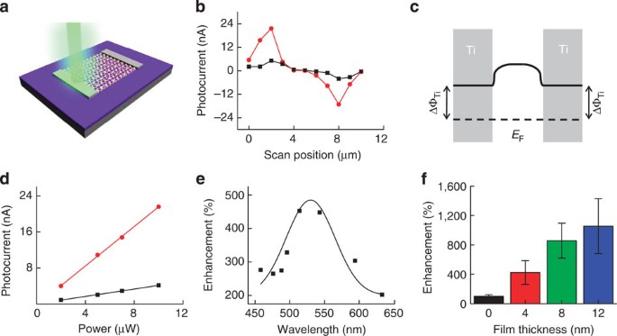Figure 3: Photocurrent measurement of the plasmon resonance enhanced graphene photodetectors. (a) Schematics of graphene photodetector, with a laser scanning across the graphene–metal (Ti) junction. All devices studied have a channel length of∼8 μm and channel width of∼8 μm. (b) Photocurrent measurement with laser scanning from outside of source electrode to the outside of drain electrode shows anti-symmetric photocurrent response. The red and black lines indicate the response of the device with and without Au nanoparticles, respectively. The electrode width is 1 μm, and the laser wavelength is 514 nm with a total power of 10 μW. (c) Band profile of the graphene photodetector. ΔΦTirepresents the difference between Dirac point energy and Fermi level in Ti-doped graphene. The Ti electrode contact slightly dopes the graphene with electrons to shift its Fermi level up towards Dirac point, and creates a potential barrier between the graphene under the electrodes and the graphene in the channel. (d) Photocurrent generated as a function of laser power. The red and black lines indicate the response of a typical device with and without Au nanoparticles, respectively. Laser wavelength is 514 nm. (e) Photocurrent enhancement as a function of laser wavelength, indicating an enhancement >400% can be observed in the devices with plasmonic Au nanoparticles, and the spectral response of the enhancement is consistent with the plasmonic resonance spectrum of the Au nanoparticles. The black squares represent the experimental data points and the solid line is the guide to the eye. (f) The photocurrent enhancement with Au nanoparticles obtained by annealing Au film of variable initial thickness (0, 4, 8 and 12 nm). With increasing Au film thickness, there is increasing plasmon resonance intensity, leading to an increased enhancement effect, with a maximum enhancement of∼1,500% observed in the device obtained from 12-nm film. The error bars show the variation of device performance from five devices. Figure 3c shows the schematic potential profile of the device, with the solid line representing graphene Dirac point and the dashed line denoting the Fermi level. Due to the smaller work function of contact metal (Ti in our case) than graphene, the graphene under the contact electrodes is a little electron doped compared with graphene in the channel, leading to a built-in potential barrier across the graphene under metal contact and the graphene in the channel. This is analogous to the traditional p-n junction photodiode, where the photo-generated electron-hole pairs can be separated by the built-in potential, contributing to the total measurable photocurrent. The built-in potential is strongest at the junction area, resulting in a maximal photocurrent detected at this position. Additionally, the same Ti contact of both electrodes can create an opposite symmetric potential profile to result in an anti-symmetrical photocurrent characteristic. Figure 3: Photocurrent measurement of the plasmon resonance enhanced graphene photodetectors. ( a ) Schematics of graphene photodetector, with a laser scanning across the graphene–metal (Ti) junction. All devices studied have a channel length of ∼ 8 μm and channel width of ∼ 8 μm. ( b ) Photocurrent measurement with laser scanning from outside of source electrode to the outside of drain electrode shows anti-symmetric photocurrent response. The red and black lines indicate the response of the device with and without Au nanoparticles, respectively. The electrode width is 1 μm, and the laser wavelength is 514 nm with a total power of 10 μW. ( c ) Band profile of the graphene photodetector. ΔΦ Ti represents the difference between Dirac point energy and Fermi level in Ti-doped graphene. The Ti electrode contact slightly dopes the graphene with electrons to shift its Fermi level up towards Dirac point, and creates a potential barrier between the graphene under the electrodes and the graphene in the channel. ( d ) Photocurrent generated as a function of laser power. The red and black lines indicate the response of a typical device with and without Au nanoparticles, respectively. Laser wavelength is 514 nm. ( e ) Photocurrent enhancement as a function of laser wavelength, indicating an enhancement >400% can be observed in the devices with plasmonic Au nanoparticles, and the spectral response of the enhancement is consistent with the plasmonic resonance spectrum of the Au nanoparticles. The black squares represent the experimental data points and the solid line is the guide to the eye. ( f ) The photocurrent enhancement with Au nanoparticles obtained by annealing Au film of variable initial thickness (0, 4, 8 and 12 nm). With increasing Au film thickness, there is increasing plasmon resonance intensity, leading to an increased enhancement effect, with a maximum enhancement of ∼ 1,500% observed in the device obtained from 12-nm film. The error bars show the variation of device performance from five devices. Full size image Comparing the photocurrent amplitude, it is obvious to notice that the graphene device with Au nanoparcticles shows an overall 4–5 times higher photocurrent than those without Au nanoparcicles. Power dependence studies show that the photocurrent scales linearly with the excitation power even at zero source-drain bias ( Fig. 3d ). The average peak photo-responsivity is about 0.42 mA W −1 for the graphene device without Au nanoparticles, comparable to previous studies at zero bias [16] , [22] . Significantly, a much larger value up to 2.2 mA W −1 is achieved for the device with the plasmonic gold nanostructures, with an average enhancement of the photoresponsivity by more than 400%. To confirm that the enhanced photoresponsivity is indeed originated from the enhanced light-trapping effect when coupled with plasmonic nanostructures, wavelength-dependent photocurrent measurement is conducted with laser focused on one of the graphene–metal junction area. After comparing with the control devices without Au nanoparticles to obtain the enhancement factors at variable wavelength, the spectral dependent response is obtained ( Fig. 3e ). Importantly, the spectral-dependent photocurrent enhancement shows an obvious peak around 530 nm, which is close to the extinction peak of graphene—nanoparticle conjugate and strongly suggests that the enhancement is indeed originated from the plasmon resonance enhanced absorption in graphene devices. In general, the photocurrent enhancement in graphene devices with Au nanoparticle array can be attributed to both the enhanced near-field oscillation and scattering effect of Au nanoparticles. Due to localized surface plasmon of gold nanoparticles, there is an oscillation of conduction electrons that arises in the metal nanoparticles when excited by a specific frequency of electromagnetic radiation. With this oscillation, light is trapped around the surface of the nanoparticles, lead to an enhanced local electrical (optical) field that can effectively enhance the total absorption of graphene. In addition, the scattering effect can also contribute to the enhanced photocurrent, similar to plasmonic enhancement effect observed in 2D nanostructure array [32] . The optical energy scattered by one nanoparticle can be collected by neighbouring nanoparticles as plasmons instead of decaying as free-space light. In this way, the plasmon oscillation of individual Au nanoparticles and the interacting scattering between neighbouring Au nanoparticles can result in a strong coupling between the nanoparticles, trapping light in the plane of the nanoparticle array and localizing optical fields on each nanoparticle, and therefore lead to a greatly enhanced optical field near graphene to dramatically enhance the overall absorption by graphene and the photocurrent. The photoresponsivity of the plasmonic-enhanced devices can be further increased by using Au nanoparticle array obtained by annealing gold thin film of increasing thickness, which can result in larger Au nanoparcticle array with increased scattering cross-section and lead to a further enhancement of local electrical field. Figure 3f shows the photocurrent enhancement of graphene devices with nanoparticles obtained from variable starting gold film thickness. Importantly, annealing 8 nm thick gold film can result in the formation of 60 nm diameter nanoparticles with a density of 76 particles per μm 2 ( Supplementary Fig. S3 ), with which on graphene an average photocurrent enhancement >800% can be achieved near graphene–metal junction; with the 110 nm-diameter nanoparticle array obtained by annealing 12 nm gold film ( Supplementary Fig. S4 ), the photocurrent can be enhanced by about 1,000% (up to 1,500% with a photoresponsivity of 6.1 mA W −1 ). These experiment results agree well with the extinction spectra of various Au nanoparticle array on graphene, in which the absorption/extinction increases significantly with increasing particle size (or the initial gold film thickness) ( Supplementary Fig. S5 ). To further understand the plasmon resonance enhanced photodetection, we have employed finite-difference time-domain technique [33] , [34] to calculate the electric field distribution near the gold nanoparticle (nanoplate) array under 514 nm incident light. The simulated electrical field distribution strongly indicates that light is enhanced and trapped in the close proximity of the nanoparticle array ( Fig. 4a–c ). We have further integrated field intensity to achieve average light intensity enhancement versus distance to the plane of nanoparticle array with different nanoparticle sizes (18, 60, 110 nm diameter) ( Fig. 4d ). The results show that the average light intensity decays rather rapidly with increasing distance from the nanoparticle plane, which is particularly evident in the smaller sized particle array. These results clearly demonstrate the importance to have a thin active layer (for example, monolayer of graphene) and to place the active layer in the close proximity of the plasmonic nanostructures to ensure maximum enhancement effect. Considering the PMMA residue between graphene and the nanoparticle array, an average enhancement factor of ∼ 4.5, ∼ 7.5 and ∼ 9.5 is achieved at a ∼ 2 nm distance from the nanoparticle plane by 18, 60 and 110 nm diameter nanoparticle array, which agrees well with the observed photocurrent enhancement. 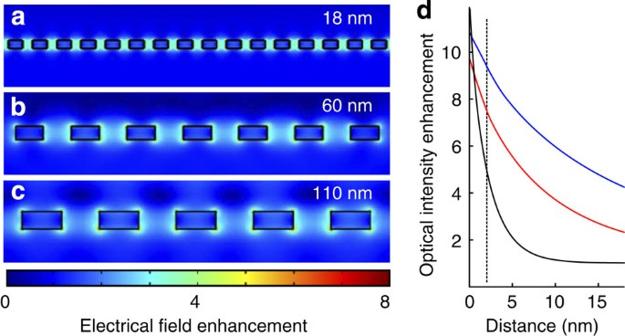Figure 4: Finite-difference time-domain (FDTD) simulation of plasmon resonance enhancement of local optical field. (a–c) Electrical field distribution near the gold nanoparticle (nanoplate) array with an average particle diameter of 18, 60 and 110 nm, respectively. The field images are cross-section of the nanoparticle array and are achieved by two-dimensional FDTD calculations. (d) Average enhanced light intensity versus distance to the plane of nanoparticle array with different nanoparticle sizes (black line for 18 nm, red line for 60 nm and blue line for 110 nm diameter). The results show that the average light intensity decays rather rapidly with increasing distance from the nanoparticle plane. Figure 4: Finite-difference time-domain (FDTD) simulation of plasmon resonance enhancement of local optical field. ( a – c ) Electrical field distribution near the gold nanoparticle (nanoplate) array with an average particle diameter of 18, 60 and 110 nm, respectively. The field images are cross-section of the nanoparticle array and are achieved by two-dimensional FDTD calculations. ( d ) Average enhanced light intensity versus distance to the plane of nanoparticle array with different nanoparticle sizes (black line for 18 nm, red line for 60 nm and blue line for 110 nm diameter). The results show that the average light intensity decays rather rapidly with increasing distance from the nanoparticle plane. Full size image Multi-colour photodetection The highly spectral selective enhancement of the photocurrent in graphene devices can readily allow us to construct multi-color photodetectors by coupling graphene with plasmonic nanostructures of designed plasmon resonance frequency. Importantly, a wide range of plasmonic nanostructures can now be readily created to exhibit distinct resonance frequencies by controlling the nanostructure size, shape and periodicity. To this end, in addition to the Au nanoparticles obtained by simple thermal anneal of Au thin films, we have created well-defined Au nanostructure array on SiO 2 /Si substrate using standard electron-beam lithography approach. These plasmonic nanostructures were then transferred onto the graphene devices using a similar process described above. In general, for the 18 nm diameter Au nanoparticles obtained by thermally annealing 4 nm thick gold film, the dark-field optical microscope image of a 50×50 μm 2 area of such nanoparticles exhibits a distinct green colour, particularly on the peripheral due to strong scattering effect and out-of-plane free-space decaying without neighbouring particles ( Fig. 5a ). This green colour in dark-field image is consistent with the ultraviolet-visible extinction spectrum obtained from such nanoparticle thin films ( Fig. 2c ). The graphene devices coupled with such nanoparticle array ( Fig. 5b ) exhibit photoresponse peak around 530 nm with a consistent maximum sensitivity to green light ( Fig. 5c ). Importantly, a well-defined array of 50 nm wide 30 nm high Au nanodisks shows yellow-green colour in the dark-field image ( Fig. 5d ), and the devices coupled with such nanodisk array ( Fig. 5e ) show an enhancement peak around 550 nm with a consistent maximum photocurrent response to a yellow-green colour ( Fig. 5f ). Further increasing the nanodisk size to 100 nm diameter in a regular array ( Fig. 5h ) leads to a more red shift in the dark-field image colour ( Fig. 5g ) with a photocurrent enhancement peak corresponding to a yellow colour detection ( ∼ 575 nm) ( Fig. 5i ). Creating rod-like Au nanostructure array ( Fig. 5k ) with orange-red dark-field image ( Fig. 5j ) can lead to even more red shift of photocurrent response to beyond 633 nm (which is our experimental limit due to the limited number lasers available in our confocal microscope) ( Fig. 5l ), resulting in a selective detection of the red-end colour. The agreement between dark-field image colour with photocurrent enhancement peak further confirms that enhanced photocurrent is a result of plasmon resonance effect of nanoparticle array. 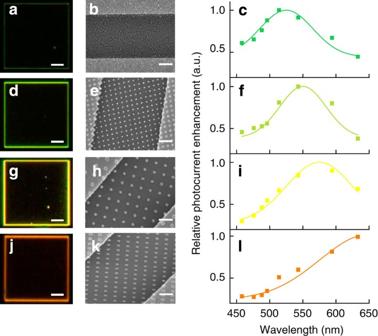Figure 5: Multi-color photodetection using graphene devices coupled with different plasmonic nanostructures. (a) Dark-field image of a 50×50 μm2area of 18 nm diameter nanoparticle array obtained by thermally annealing 4 nm Au thin film. (b) Scanning electron microscopy (s.e.m.) image of a representative device with the nanoparticle array, and (c) the corresponding spectral response of the photocurrent enhancement. (d) Dark-field image of a 50×50 μm2area of 50 nm diameter 30-nm height nanodisk array. (e) s.e.m. image of a representative device with the 50-nm diameter nanodisk array, and (f) the corresponding spectral response of the photocurrent enhancement. (g) Dark-field image of a 50×50 μm2area of 100 nm diameter 30 nm height nanodisk array. (h) SEM image of a representative device with the 100-nm diameter nanodisk array, and (i) the corresponding spectral response of the photocurrent enhancement. (j) Dark-field image of a 50×50 μm2area of 100 nm length, 50 nm width and 30-nm height nanorod array. (k) SEM image of a representative device with the nanorod array, and (l) the corresponding spectral response of the photocurrent enhancement. Scale bars are 10 μm ina,d,gandjand 400 nm inb,e,handk. The plasmonic nanostructures ind,gandjare obtained by using e-beam lithography to define Au patterns. The square symbols and the lines inc,f,iandlrepresent the experimental data points and the line guide to the eye. The photocurrent measurement is obtained by focused laser illumination of the grahene–metal contact of the graphene device with∼8 μm channel length and 8 μm channel width. The spectral response of graphene devices is consistent with the dark-field image colour of the corresponding plasmonic nanostructures, further confirming the plasmonic enhancement effect and demonstrating that the multi-color photodetection can be achieved by coupling the graphene devices with plasmonic nanostructures of different resonance features. Figure 5: Multi-color photodetection using graphene devices coupled with different plasmonic nanostructures. ( a ) Dark-field image of a 50×50 μm 2 area of 18 nm diameter nanoparticle array obtained by thermally annealing 4 nm Au thin film. ( b ) Scanning electron microscopy (s.e.m.) image of a representative device with the nanoparticle array, and ( c ) the corresponding spectral response of the photocurrent enhancement. ( d ) Dark-field image of a 50×50 μm 2 area of 50 nm diameter 30-nm height nanodisk array. ( e ) s.e.m. image of a representative device with the 50-nm diameter nanodisk array, and ( f ) the corresponding spectral response of the photocurrent enhancement. ( g ) Dark-field image of a 50×50 μm 2 area of 100 nm diameter 30 nm height nanodisk array. ( h ) SEM image of a representative device with the 100-nm diameter nanodisk array, and ( i ) the corresponding spectral response of the photocurrent enhancement. ( j ) Dark-field image of a 50×50 μm 2 area of 100 nm length, 50 nm width and 30-nm height nanorod array. ( k ) SEM image of a representative device with the nanorod array, and ( l ) the corresponding spectral response of the photocurrent enhancement. Scale bars are 10 μm in a , d , g and j and 400 nm in b , e , h and k . The plasmonic nanostructures in d , g and j are obtained by using e-beam lithography to define Au patterns. The square symbols and the lines in c , f , i and l represent the experimental data points and the line guide to the eye. The photocurrent measurement is obtained by focused laser illumination of the grahene–metal contact of the graphene device with ∼ 8 μm channel length and 8 μm channel width. The spectral response of graphene devices is consistent with the dark-field image colour of the corresponding plasmonic nanostructures, further confirming the plasmonic enhancement effect and demonstrating that the multi-color photodetection can be achieved by coupling the graphene devices with plasmonic nanostructures of different resonance features. Full size image These studies clearly demonstrate that spectral selective multi-color photodetection can be readily achieved by coupling graphene photodetector with different plasmonic nanostructures. With this approach, it is possible to integrate multicolour photosensor pixels in a small footprint as little as a few square micrometres or less, and therefore enable a new generation of high performance, high speed, high resolution, low cost and zero operation voltage (zero dark current) photosensor arrays for a wide range of applications ranging from imaging cameras to optical communication devices. Plasmon resonance enhanced photodetection in asymmetric devices With the same metal contact on both electrodes in the metal-graphene-metal device, the potential profile is symmetric within the channel and the photocurrent is antisymmetric and opposite near both metal-graphene contacts, leading to a zero total current if device is illuminated globally. To this end, asymmetric metal electrodes can be employed to break the mirror symmetry in band profile to allow the observation of an overall photocurrent in the device, as demonstrated in a recent study [22] . For example, metal of different work functions (for exampe, Ti and Pd, ref. 22 ) can be used as the different contact material ( Fig. 6a ). In this case, the photocurrent generated near the Ti electrode side is identical with Ti-contacted symmetric device ( Fig. 3 ). The difference exists at the Pd electrode side, where the high work function of Pd cause nearly no additional doping to the underneath graphene and a nearly flat band structure is formed around this electrode with the expectation of little photocurrent (inset, Fig. 6b ). Indeed, scanning photocurrent measurement conducted under zero bias and zero gate voltage shows that photocurrent can only be observed near the Ti contact side, but not Pd side ( Fig. 6b ). Similarly, compared with the control device without Au nanoparticles (black line), our plasmonic enhanced device (with 18 nm particle array) exhibits a >400% enhancement, consistent with the symmetric devices discussed above ( Fig. 3 ). The global illumination measurement is conducted using a defocused 532 nm green laser to cover the whole device. 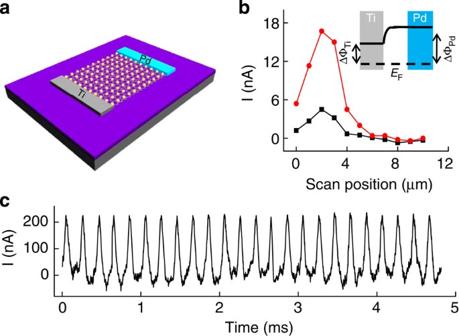Figure 6: Plasmon resonance enhanced graphene photodetectors with asymmetric metal contacts. (a) Schematic illustration of a graphene photodetector with asymmetric metal contacts (Ti and Pd) that can enable photocurrent generation under global illumination. (b) Photocurrent profile with laser scanning from outside of Ti electrode (black line: normal graphene device; red line: plasmon resonance enhanced graphene device). The inset shows the band profile of asymmetric metal-contacted graphene photodetector. ΔΦTiand ΔΦPdrepresent the difference between Dirac point energy and Fermi level in Ti-doped graphene and Pd-doped graphene, in which Ti raises the Fermi-level energy position, whereas Pd maintains nearly the original Fermi level position of the intrinsically p-doped graphene. The photocurrent can only be seen with illumination near the Ti electrodes because bend bending only occurs there. (c) Time-dependent photocurrent measurement with a global laser (532 nm) illumination through a 5.2 kHz chopper. Figure 6c shows the overall photocurrent of the asymmetrical device obtained under global illumination with a 5.2 kHz mechanical chopper in front of laser. The periodic photoresponse characteristics exhibit the same frequency as that of the mechanical chopper, clearly demonstrating the generation of overall photocurrent in the asymmetric device in response to global illumination. Figure 6: Plasmon resonance enhanced graphene photodetectors with asymmetric metal contacts. ( a ) Schematic illustration of a graphene photodetector with asymmetric metal contacts (Ti and Pd) that can enable photocurrent generation under global illumination. ( b ) Photocurrent profile with laser scanning from outside of Ti electrode (black line: normal graphene device; red line: plasmon resonance enhanced graphene device). The inset shows the band profile of asymmetric metal-contacted graphene photodetector. ΔΦ Ti and ΔΦ Pd represent the difference between Dirac point energy and Fermi level in Ti-doped graphene and Pd-doped graphene, in which Ti raises the Fermi-level energy position, whereas Pd maintains nearly the original Fermi level position of the intrinsically p-doped graphene. The photocurrent can only be seen with illumination near the Ti electrodes because bend bending only occurs there. ( c ) Time-dependent photocurrent measurement with a global laser (532 nm) illumination through a 5.2 kHz chopper. Full size image To further probe the plasmon resonance enhancement effect and overall device performance, it is important to determine the overall external QE of the device at zero bias. For the control graphene device without the Au nanoparticles, the photo-responsivity is about 0.4 mA W −1 at 514 nm, which translates to an external QE of 0.1%, and is comparable to the external QE observed in previously reported graphene photodetectors ( ∼ 0.1–0.2% at zero bias) [16] , [22] . Importantly, for the graphene device with Au nanoparticles, the maximum photoresponsivity can reach up to 6.1 mA W −1 at 514 nm with an external QE of ∼ 1.5%, which is more than one order of magnitude increase over the device without the plasmonic nanostructures under similar bias conditions. Such a high plasmonic enhancement effect is rarely observed in traditional planar semiconductor devices [35] because the local enhancement nature of plasmonic resonance can only affect semiconductor material in the very proximity of the plasmonic nanostructures (for example, decay length within ∼ 10 nm, Fig. 4 ) [36] , while the active depth of the traditional semiconductor device is usually much bigger. With the nature of a single atomic thickness, the entire graphene can be placed within the close proximity of the plasmonic nanostructures and therefore it can fully exploit the local plasmonic enhancement effect to achieve an unprecedented enhancement not possible with other planar semiconductors. It is also important to note that all our results discussed above were obtained at zero gate voltage and zero source drain bias to pursue zero power consumption photodetectors. The QE can be further improved by tuning the gate voltage ( Supplementary Fig. S6 ), contact metals and/or source-drain bias to optimize the graphene–metal potential barrier [22] . In addition to the built-in electrical potential near the graphene–metal contact, photothermoelectric effect has also been reported to have an important role in photocurrent generation [37] , which could contribute to the observed photocurrent in our devices as well. Nonetheless, regardless of the exact mechanism for photocurrent generation, the enhancement of local optical field by coupling with plasmonic nanostructures would produce a similar effect to amplify the overall photoresponsivity of the graphene photodetectors. In summary, we have demonstrated a new concept of highly specific multi-color graphene photodetectors by coupling graphene devices with plasmonic nanostructures. Coupling plasmonic thin film with the atomic thin graphene creates a greatly enhanced local optical field near the graphene plane, and result in an overall plasmonic enhancement by more than a factor of 10. With this substantial enhancement and further optimization of the device structures to improve built-in potential and the active area [22] , a further enhancement of the overall photoresponsivity can be expected. Together with demonstrated abilities including zero operation voltage, high speed, flexibility and ultra-wide band absorption, the scalable fabrication of plasmon resonance enhanced graphene photodetectors can open up exciting opportunities for future graphene-based optoelectronics. Last, coupling the atomically thin graphene with plasmonic nanostructures can most effectively convert local plasmonic enhancement effect into electrical signal to enable fast direct electrical read-out of plasmonic resonance, and thus has the potential to enable the design of a new generation of plasmon resonance-based devices for image sensor array or multiplexed bio-sensor array [38] , [39] . During the review process, we became aware of another work on a similar topic [40] . Our study was developed independently. Graphene growth and transfer The graphene was grown by CVD on copper foil at 1,050 °C with methane as the carbon-containing precursor. At first, Cu foils (25 μm thick, 99.8%, Alfa Aesar) were loaded into a 1-inch quartz tube inside a horizontal furnace of a commercial CVD system. The furnace is then allowed to heat up to 1,080 °C with H 2 /Ar flow (25 sccm/475 sccm) to anneal the Cu foil for 90 min. After annealing, the temperature is dropped to 1,050 °C in 10 min. The graphene growth was initiated by feeding methane (500 p.p.m. methane in Ar, 35 sccm) balanced with the H 2 /Ar (25 sccm/440 sccm). After growth, the graphene was transferred onto silicon/silicon oxide substrate for characterization and device fabrication. Initially, the graphene was grown on both sides of the copper foils. To transfer the graphene, we first spin coated a layer of PMMA film onto one side of the graphene/Cu foil and clean the other side with O 2 plasma. The copper is then etched away using copper etchant by floating the foil on the surface of the etchant bath. The PMMA/graphene film is washed with HCl/H 2 O (1:10) and DI water for several times, and transferred onto silicon/silicon oxide or glass substrate. Graphene device fabrication and characterization Photolithography process was used to pattern graphene into 8×20 μm blocks on silicon/silicon oxide (300 nm SiO 2 ) substrate. Source-drain electrodes (Ti/Au: 50 nm/50 nm) were then defined by standard E-beam lithography technique followed by E-beam deposition to result in back-gated graphene transistors. The gold nanoparticle thin film was prepared and transferred onto graphene as described in the main text. The transport characteristics measurements were conducted with a probe station and a computer-controlled analogue-to-digital converter at room temperature. The ultraviolet-visible extinction measurement was conducted using Beckman-Coulter DU-800 spectrophotometer (Beckman-Coulter) with wavelength ranging from 400 nm to 700 nm range. Raman spectrum experiments are carried out using Renishaw inVia Raman microscope (Renishaw). The measurement is conducted under 514 nm Ar laser with a spot size around 1 μm. Scanning photocurrent measurement is conducted using DL 1211 low-noise current preamplifier and a computer-controlled analogue-to-digital converter, with a SP2 MP Film confocal microscope coupled with Ar/ArKr laser (wavelength 458, 476, 488, 496 and 514 nm) and HeNe laser (543, 596 and 633 nm). How to cite this article: Liu Y. et al . Plasmon resonance enhanced multicolour photodetection by graphene. Nat. Commun. 2:579 doi: 10.1038/ncomms1589 (2011).